Spin current generated by thermally driven ultrafast demagnetization Spin current is the key element for nanoscale spintronic devices. For ultrafast operation of such nano-devices, generation of spin current in picoseconds, a timescale that is difficult to achieve using electrical circuits, is highly desired. Here we show thermally driven ultrafast demagnetization of a perpendicular ferromagnet leads to spin accumulation in a normal metal and spin transfer torque in an in-plane ferromagnet. The data are well described by models of spin generation and transport based on differences and gradients of thermodynamic parameters. The temperature difference between electrons and magnons is the driving force for spin current generation by ultrafast demagnetization. On longer timescales, a few picoseconds following laser excitation, we also observe a small contribution to spin current by a temperature gradient and the spin-dependent Seebeck effect. The field of spintronics is concerned with efficient generation of spin currents and control of magnetic elements. Conventionally, spin currents are generated by passing electrical currents through ferromagnetic materials [1] , [2] , [3] , [4] , [5] . Recently, much effort has been expended to understand the generation of spin currents by thermal gradients [6] , [7] , [8] , [9] , [10] , [11] , [12] , [13] , [14] . Yet, another route to generate spin currents is rapid demagnetization of a ferromagnetic layer by direct excitation with an ultrashort laser pulse. Ultrafast demagnetization by an ultrashort laser pulse has been investigated extensively in recent years [15] , [16] , [17] , [18] , [19] , and has been described by a three-temperature model [15] wherein the electronic, magnon and phonon excitations are characterized by three separate temperatures. The three-temperature model considers energy conservation, but the relaxation mechanism of spin angular momentum is controversial. Koopmans et al. [19] explained rapid demagnetization by electron–phonon-mediated spin-flip scattering. Battiato et al. [20] proposed that spin-dependent relaxation and fast transport of hot electrons play a crucial role and suggested that ultrafast demagnetization produces spin-polarized hot electrons, which move to an adjacent metallic layer by a so-called ‘superdiffusive current’. The findings of several subsequent experiments have been interpreted as supporting this hypothesis [21] , [22] , [23] , [24] , [25] . However, the superdiffusive model is based on non-thermal electronic motion [20] and the transport of thermal energy is not considered in these experiments [21] , [22] , [23] , [24] , [25] . Recently, we have shown that the exchange of thermal energy between metal layers is crucial in the interpretation of demagnetization of a ferromagnet (FM) in a metallic multilayer structure [26] . Therefore, we argue that a comprehensive analysis of the exchange of thermal energy in the system and the implementation of a direct method for detecting demagnetization-induced spin currents is needed. In the following, we show that deviations from thermodynamic equilibrium can be used to describe the mechanism for spin current generation induced by demagnetization. There are three aspects to our experiments. First, we measure the demagnetization of an FM sandwiched between two normal metals (NMs) and analyse thermal transport in the sample to explain the demagnetization. Second, we measure the demagnetization-induced spin accumulation in the NM and provide an analysis of diffusive spin transport to explain the spin accumulation. Third, we measure the demagnetization-induced spin transfer torque (STT) using an NM/FM1/NM/FM2 structure where the second magnetic layer FM2 has magnetization that is perpendicular to FM1. Previously, the generation of STT has been realized by an electric field [1] , [2] , [3] , [4] , [5] or a temperature-gradient [6] , [7] applied across the sample. Here we show an alternative method for generating STT using ultrafast demagnetization. Experiment We prepared two types of ferromagnetic structures. The first type consists of, essentially, Pt (30 nm)/FM1/Cu ( h nm) (we refer to this as the Cu- h nm sample), and the second type consists of Pt (30 nm)/FM1/Cu (10 nm)/FM2 (2 nm) (we refer to this as the CoFeB-2 nm sample). FM1 is a FM with perpendicular magnetization ([Co (0.5 nm)/Pt (1 nm)] × 4 /Co (0.5) or [Co (0.4 nm)/Pt (1 nm)] × 4 /Co (0.2 nm)/Ni (0.4 nm)/Co (0.2) multilayer) and FM2 is an ferromagnetic CoFeB layer with in-plane magnetization (see Methods for a detailed description of the sample preparation). The concept of how we generate a spin current from demagnetization is shown schematically in Fig. 1 . The pump laser pulse excites the Pt layer and leads to the demagnetization of FM1 by thermal transport from Pt to FM1. The ultrafast demagnetization of FM1 generates a spin current by electron–magnon coupling in FM1, as we will justify below, and by diffusive spin transport. This spin current accumulates in the Cu layer in the first type of structure and is absorbed by FM2 in the second type of structure. In the second type of structure, the FM1 layer has out-of-plane magnetization, whereas the FM2 layer has in-plane magnetization. This perpendicular configuration is an effective way for observing magnetization dynamics due to the spin current-induced STT; although thermal fluctuations of magnetization yield non-zero STT even for collinear magnetic configurations, the observation of STT effect in a collinear configuration requires a threshold of spin current to trigger magnetization dynamics [4] , while the transverse STT does not. 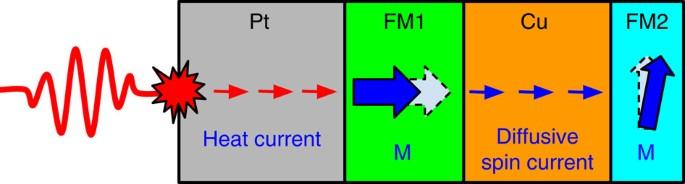Figure 1: Conceptual diagram. Pump laser is incident on 30-nm-thick Pt side and creates an ultrafast temperature excursion. Thermal transport from Pt to FM1 ([Co/Pt]) drives demagnetization of the perpendicular ferromagnetic layer FM1. The demagnetization of FM1 generates a diffusive spin current in the adjacent Cu layer that is absorbed by the in-plane ferromagnetic layer FM2 (CoFeB). STT tilts the magnetization of FM2 out of plane and the magnetization of FM2 begins to precess. Figure 1: Conceptual diagram. Pump laser is incident on 30-nm-thick Pt side and creates an ultrafast temperature excursion. Thermal transport from Pt to FM1 ([Co/Pt]) drives demagnetization of the perpendicular ferromagnetic layer FM1. The demagnetization of FM1 generates a diffusive spin current in the adjacent Cu layer that is absorbed by the in-plane ferromagnetic layer FM2 (CoFeB). STT tilts the magnetization of FM2 out of plane and the magnetization of FM2 begins to precess. Full size image We apply a laser pulse on the Pt side of the samples for two reasons. The first reason is to minimize the contribution from hot electron transport with excess energy on the order of the photon energy [20] . The inelastic mean-free path of hot electrons in Pt is ≈5 nm [27] . As the [Co/Pt] multilayer is indirectly heated by a relatively thick Pt layer (30 nm), the strong electron–electron and electron–phonon scattering in Pt (ref. 28 ) should greatly suppress the density of hot electrons that reach the [Co/Pt] layer. When the density of far-from equilibrium hot electrons is negligible in the [Co/Pt] layer, the superdiffusive model [20] does not predict the demagnetization or a demagnetization-induced spin current. Eschenlohr et al. [24] reported that Ni has a comparable demagnetization whether it is excited directly by laser pulse or indirectly through a Au layer. This result can be interpreted, as indicating that the superdiffusive model is applicable even when hot electrons transport through the Au layer. However, we have shown that weak electron–phonon coupling of Au and fast electronic transport across the Au/Ni interface can explain the observations as well [26] . The second reason is to moderate the initial change of the magnetization of the CoFeB layer, which may be important to estimate spin angular momentum transfer efficiency based on the STT theory established for a single domain state [1] , [2] , [29] . Substantial demagnetization of CoFeB accompanied by the simultaneous arrival of a transverse spin current may prevent us from applying the STT theory. We use time-resolved measurements of the polar magneto-optical Kerr effect (TR-MOKE) to detect the transient magnetic and spin signals in the film-normal direction. We (i) measured the demagnetization of the [Co/Pt] layer with the probe beam on the Pt side of the Cu- h nm samples; (ii) measured the spin accumulation of the Cu layer with the probe beam incident on the Cu side of the Cu- h nm samples; and (iii) measured the precession of the CoFeB layer with the probe beam on the CoFeB side of the CoFeB-2 nm sample. In separate experiments, we use time-domain thermoreflectance (TDTR) to measure the temperature excursion of the Pt or Cu layers (see Methods for further details of the measurement techniques). Demagnetization of the [Co/Pt] layer When both pump and probe beams are incident on the Pt side of the Cu-80 nm sample, we observe a rapid demagnetization of the [Co/Pt] layer on a sub-picosecond timescale and partial recovery of the magnetization that is complete after a few picoseconds ( Fig. 2a ). The peak change in the Kerr rotation due to the rapid demagnetization is −9.6±1 μrad at 0.5 ps. We compare this value with the static Kerr rotation, 116±10 μrad that we measure for the Cu-80 nm sample. Based on linear scaling of Kerr rotation with magnetization, we conclude that a pump fluence of 17 J m −2 , which results in an absorbed fluence of 6 J m −2 (see Supplementary Note 1 ), creates a maximum change of magnetization of at 0.5 ps and a net change of magnetization of after 3 ps. 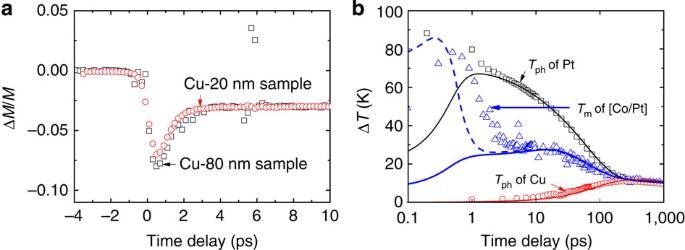Figure 2: Demagnetization of the [Co/Pt] layer. (a) Demagnetization of the [Co/Pt] layer of the Cu-80 nm sample measured with the probe beam on the Pt side (black square) and that of the Cu-20 nm sample with probe beam on the Cu side (red circle). Normalizing with static Kerr rotation, the relative change in magnetizationΔM/Mis −0.08±0.02 and −0.07±0.02, respectively, at 0.5 ps with the same pump fluence of 17.3 J m−2. The peak observed at 6 ps is an artefact due to coherent interference between the pump and probe light due to a stray reflection. (b) The result of thermal analysis. Pt phonon temperature from a TDTR measurement on the Pt side (black square), Cu phonon temperature from a TDTR measurement on the Cu side (red circle) and [Co/Pt] magnon temperature from MOKE measurement on the Pt side (blue triangle). Solid and dotted lines are results of thermal modelling; black solid line is for Pt phonon temperatures; red solid line is for Cu phonon temperatures; blue solid line is for [Co/Pt] phonon temperatures; blue dotted line is for [Co/Pt] electron temperatures. The thermal modelling is done by solving heat diffusion equations of Pt/[Co/Pt]/Cu structure (seeSupplementary Note 4for details about thermal modelling). Figure 2: Demagnetization of the [Co/Pt] layer. ( a ) Demagnetization of the [Co/Pt] layer of the Cu-80 nm sample measured with the probe beam on the Pt side (black square) and that of the Cu-20 nm sample with probe beam on the Cu side (red circle). Normalizing with static Kerr rotation, the relative change in magnetization ΔM / M is −0.08±0.02 and −0.07±0.02, respectively, at 0.5 ps with the same pump fluence of 17.3 J m −2 . The peak observed at 6 ps is an artefact due to coherent interference between the pump and probe light due to a stray reflection. ( b ) The result of thermal analysis. Pt phonon temperature from a TDTR measurement on the Pt side (black square), Cu phonon temperature from a TDTR measurement on the Cu side (red circle) and [Co/Pt] magnon temperature from MOKE measurement on the Pt side (blue triangle). Solid and dotted lines are results of thermal modelling; black solid line is for Pt phonon temperatures; red solid line is for Cu phonon temperatures; blue solid line is for [Co/Pt] phonon temperatures; blue dotted line is for [Co/Pt] electron temperatures. The thermal modelling is done by solving heat diffusion equations of Pt/[Co/Pt]/Cu structure (see Supplementary Note 4 for details about thermal modelling). Full size image When the Cu layer is sufficiently thin, the demagnetization of the [Co/Pt] layer can also be detected by probing from the Cu side. With the Cu-20 sample, we obtain following the same approach as described above. When probing from the Cu side of the sample, the peak of the transient Kerr rotation decreases exponentially with increasing Cu layer thickness (see Supplementary Note 2 and Supplementary Fig. 1 ). This is because the Kerr rotation generated directly by the magneto-optic properties of the [Co/Pt] layer is attenuated by the small optical transmission of thick Cu layers. In what follows, we focus on measurements of spin accumulation in the Cu layers of thickness h >80 nm, where the transient Kerr rotation generated directly by the change in the magnetization of the [Co/Pt] layer is small. We adopt the viewpoint that demagnetization is a result of excitation of magnons [15] , [30] , [31] and explain the demagnetization of the [Co/Pt] layer by the exchange of thermal energy between electrons, magnons and phonons, see Fig. 2b . As the [Co/Pt] layer is indirectly heated by the Pt layer, we consider thermal energy transport from the Pt layer, through the [Co/Pt] layer, and into the Cu layers. We measure the temperature of each layer independently: TDTR on the Pt side for the Pt phonon temperature, TDTR on the Cu side for the Cu phonon temperature and TR-MOKE on the Pt side for the [Co/Pt] magnon temperature (see Supplementary Note 3 for details of the TDTR measurements). Next, we model the thermal transport by numerically solving coupled heat diffusion equations of Pt/[Co/Pt]/Cu structure that describe the transport of thermal energy by electrons and phonons in each layer (see Supplementary Note 4 for details of the thermal modelling). At 0.2 ps, the electron temperature, T e , of the [Co/Pt] layer (blue dotted line) sharply increases by Δ T ≈90 K due to electronic thermal transport from the Pt layer. Owing to electron–magnon coupling of [Co/Pt], the magnon temperature, T m (blue triangle symbol), increases by ≈80 K at 0.5 ps. (We attribute this small difference in the peak temperature of electron and magnon to the uncertainty of defining zero time delay in experiment; for the modelling, we set the zero time delay to the middle of pulse light; for the measurement, we set the zero time delay to the midpoint of the initial rise of the TDTR signal generated by Pt.) Although refs 15 , 30 use the term ‘spin temperature’ to describe the temperature of the magnon system, we prefer the term ‘magnon temperature’, because ‘spin temperature’ is sometimes used to refer to the temperature of spin-up or spin-down electrons. A temperature excursion of the magnon system of Δ T m ≈80 K agrees with our observation of Δ M / M =−0.08 based on the previously reported temperature-dependent magnetization of [Co/Pt] [32] . After 1 ps, the electron temperature equilibrates with the phonon temperature, T ph , of the [Co/Pt] layer (blue solid line), and the magnon temperature and magnetization partially recovers. To model the spin current generation, we assume that electron–magnon coupling conserves spin angular momentum [30] . Thus, the spin loss by demagnetization should be converted to spin generation, that is, spin polarization in the electrons, and the spin generation rate is the negative of the demagnetization rate, − dM / dt (see Supplementary Note 5 ). In contrast to the superdiffusive model [20] , our modelling is a thermal description of demagnetization-induced spin generation: the temperature difference between electron and magnon drives flows of energy and spin angular momentum. To model this effect, we include conservation of spin angular momentum in the conventional three-temperature model [15] . 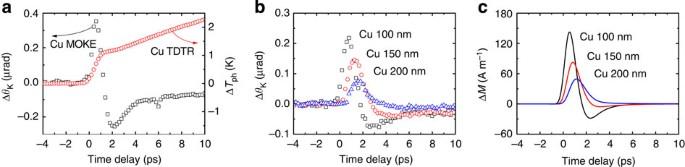Figure 3: Spin accumulation on the Cu layer. (a) TR-MOKE data (black square) and TDTR data (red circle) of the Cu-80 nm sample with the probe beam on the Cu side at pump fluence of 36 J m−2. Here we use two times larger pump fluence to increase signal-to-noise ratio. (b) Kerr rotation of Cu-100, Cu-150 and Cu-200 nm samples at pump fluence of 36 J m−2(back square for Cu-100 nm, red circle for Cu-150 nm and blue triangle for Cu-200 nm). The positive Kerr rotation of the Cu-80 nm sample is 1.6 times larger than that of Cu-100 nm sample. Given the similar Cu thickness, we expect this increase is due to the inclusion of the Co/Ni layer in Cu-80 nm sample (see Methods). (c) The spin accumulation at the end of the Cu layer obtained by solving coupled diffusion equation of Pt (30)/[Co/Pt] (6.5)/Cu (100∼200) structure at pump fluence of 17 J m−2; black solid line is for Cu-100 nm; red solid line is for Cu-150 nm; blue solid line is for Cu-200 nm. Spin accumulation in the Cu layer Figure 3 shows the transient Kerr rotation signal in the Cu layer, probed on the Cu side of the Cu-80 nm sample. A relatively sharp positive-going Kerr rotation is followed by a broader negative-going one ( Fig. 3a,b ). As the demagnetization of the [Co/Pt] layer itself produces a negative Kerr rotation (see Fig. 2a ), we conclude that the positive Kerr rotation signal is caused by spin accumulation in the Cu layer. Figure 3: Spin accumulation on the Cu layer. ( a ) TR-MOKE data (black square) and TDTR data (red circle) of the Cu-80 nm sample with the probe beam on the Cu side at pump fluence of 36 J m −2 . Here we use two times larger pump fluence to increase signal-to-noise ratio. ( b ) Kerr rotation of Cu-100, Cu-150 and Cu-200 nm samples at pump fluence of 36 J m −2 (back square for Cu-100 nm, red circle for Cu-150 nm and blue triangle for Cu-200 nm). The positive Kerr rotation of the Cu-80 nm sample is 1.6 times larger than that of Cu-100 nm sample. Given the similar Cu thickness, we expect this increase is due to the inclusion of the Co/Ni layer in Cu-80 nm sample (see Methods). ( c ) The spin accumulation at the end of the Cu layer obtained by solving coupled diffusion equation of Pt (30)/[Co/Pt] (6.5)/Cu (100 ∼ 200) structure at pump fluence of 17 J m −2 ; black solid line is for Cu-100 nm; red solid line is for Cu-150 nm; blue solid line is for Cu-200 nm. Full size image Figure 3a demonstrates that the timescale of the positive-going Kerr signal coincides with initial rise time of the TDTR signal. The TDTR signal is mostly controlled by T ph of Cu; T ph increases rapidly on short timescales because of fast energy transport by electronic excitations that are initially out of equilibrium with the Cu phonons. In other words, the Kerr rotation measures the non-equilibrium spin population in the Cu layer and the TDTR signal measures an integral of how much energy has been deposited into the phonon system by electronic thermal diffusion. From the data plotted as Fig. 3b , we observe that the time delay corresponding to the position of the positive-going peak of Kerr rotation increases with increasing Cu thickness. The spin propagation velocity is on the order of 100 nm ps −1 , much lower than Fermi velocity ( ∼ 1,600 nm ps −1 ) of Cu, suggesting that the spin currents we observe are mostly diffusive. To further understand the origin of the positive and negative peaks shown in Fig. 3b , we conduct numerical simulations of time-dependent spin transport. We use a diffusive model to describe spin accumulation in the Cu layer because we expect that ballistic hot electrons are effectively suppressed by the relatively thick Pt layer in our experiment. The spin diffusion equation is as follows [33] , [34] , where μ s =μ ↑ −μ ↓ is the spin chemical potential, D is the spin diffusion constant and τ S is the spin relaxation time. The diffusion constants of Pt and [Co/Pt] are 200 and 100 nm 2 ps −1 , respectively, calculated by , where Λ e is the electronic thermal conductivity and C e is the electronic heat capacity (see Supplementary Table 1 ). The spin relaxation time of Pt is set to 0.5 ps using , where l S is the spin diffusion length; l S =10 nm in Pt (ref. 35 ). For Cu, D =6,500 nm 2 ps −1 and τ S =25 ps (ref. 36 ). The τ S of [Co/Pt] has not been reported; hence, we use as an estimate , where τ 0 is the momentum relaxation time and a sf is the spin-flip probability from theory of Elliot–Yafet [37] , [38] . The τ 0 of [Co/Pt] is calculated to be 5 fs using , where v F is the Fermi velocity; v F =0.24 × 10 6 m s −1 for Pt [111] direction [39] . The a sf of typical ferromagnetic transition metals is 0.1 ∼ 0.2 (ref. 19 ) and that of Co has been calculated to be 0.01 ∼ 0.02 (ref. 40 ). Considering multiple interfaces of the [Co/Pt] layer, we use a sf =0.1 and τ 0 =5 fs; the τ S of [Co/Pt] is then 0.05 ps. Although τ S determined in this way has large uncertainties, we find τ S =0.05 ps of [Co/Pt] agrees with the STT result described below. We solve the coupled diffusion equations for Pt (30)/[Co/Pt] (6.5)/Cu (100 ∼ 200) structures by equating the spin chemical potential at the interfaces. (We do not include a finite spin conductance in this modelling, which we will use later in analysing the STT experiment, because we found that a finite spin conductance does not significantly change the predicted spin accumulation in these relatively thick Cu layers.) We include the spin generation term in the [Co/Pt] layer by assuming that the spin generation rate is − dM/dt ; dM/dt is obtained by numerical differentiation of the demagnetization data shown in Fig. 2a (see Supplementary Fig. 2 ). The predicted spin accumulation at the end of the Cu layer with different Cu thickness is shown in Fig. 3c . The overall time-dependent behaviour is in excellent agreement with that of the transient Kerr rotation ( Fig. 3b ). For example, the broad negative peak following the positive peak is reproduced by our model of spin diffusion, implying that diffusive spin transport and spin generation by ultrafast demagnetization captures the key features of the time-dependent spin accumulation in the Cu layer. This result supports our assumption that we can describe spin generation and spin transport in our samples in terms of differences and gradients in thermodynamic parameters. Spin current by a temperature gradient However, we also observe an important difference between the model and the experiment at delay times beyond a few picoseconds. The measured Kerr signal does not decay to zero at 10 ps, whereas the calculated spin accumulation does decay to zero. We attribute this small signal at long delay times to a spin current generated by the temperature gradient of the [Co/Pt] layer. The ultrashort light pulse produces not only a temperature difference between different heat reservoirs (electrons, magnons and phonons) but also differences in temperatures at different locations in the sample. Slachter et al. [8] showed that a steady temperature gradient in NiFe produces spin current at the NiFe/Cu interface due to the spin-dependent Seebeck effect. Following the analysis of ref. 8 , the spin current, J S , is related to the the spatial temperature gradient by, where μ B is the Bohr magneton, e is the elementary charge, σ ↑,↓ is the spin-dependent electric conductivity, S ↑,↓ is the spin-dependent Seebeck coefficient and ∇ T is the electronic temperature gradient. The spin-dependent Seebeck coefficient leads to an abrupt change of spin current going from FM to NM and thereby generates spin current at the Pt/[Co/Pt] and [Co/Pt]/Cu interfaces with opposite sign [8] . We analyse the Cu-200 nm sample to make sure that the demagnetization signal of [Co/Pt] is completely suppressed by a thick Cu layer (see Supplementary Note 2 ). In Fig. 4a , we estimate the time dependence of the temperature gradient ∇ T ( t ) of the [Co/Pt] layer from the analysis of thermal transport in the sample described above. With this ∇ T and σ =2.7 × 10 6 Ω −1 m −1 , which is obtained by applying Wiedemann–Franz law to the thermal conductivity of the [Co/Pt] layer, we calculate the ∇ T -driven spin accumulation of the Cu-200 nm sample using our spin diffusion modelling. By comparing the experimental Kerr rotation and the predicted spin accumulation, see Fig. 4b,c , we obtain a best fit to the data using . 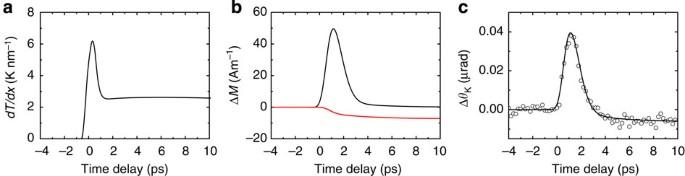Figure 4: Spin current by spatial temperature gradient. (a) Estimation of the electronic temperature gradient of [Co/Pt] in the Cu-200 nm sample from the thermal analysis. (b) Estimation of the spin accumulation at the end of Cu layer of Cu-200 nm sample with the∇T-driven spin current (red solid line). For comparison, the black solid line is the spin accumulation due to the demagnetization-induced spin current inFig. 3c. All calculations are done with a pump fluence of 17 J m−2. (c) Comparison between the spin accumulation data (black circle) and the simulated result (black solid line) of the Cu-200 nm sample with a pump fluence of of 17 J m−2. The spin accumulation data is taken fromFig. 3band divided by a factor of two because the data is obtained with a pump fluence of 35 J m−2. The time delay of the data has been shifted to −0.4 ps for matching with the simulation. The simulation result (black solid line) is the sum of black solid line and red solid line ofb. Figure 4: Spin current by spatial temperature gradient. ( a ) Estimation of the electronic temperature gradient of [Co/Pt] in the Cu-200 nm sample from the thermal analysis. ( b ) Estimation of the spin accumulation at the end of Cu layer of Cu-200 nm sample with the ∇ T -driven spin current (red solid line). For comparison, the black solid line is the spin accumulation due to the demagnetization-induced spin current in Fig. 3c . All calculations are done with a pump fluence of 17 J m −2 . ( c ) Comparison between the spin accumulation data (black circle) and the simulated result (black solid line) of the Cu-200 nm sample with a pump fluence of of 17 J m −2 . The spin accumulation data is taken from Fig. 3b and divided by a factor of two because the data is obtained with a pump fluence of 35 J m −2 . The time delay of the data has been shifted to −0.4 ps for matching with the simulation. The simulation result (black solid line) is the sum of black solid line and red solid line of b . Full size image We also determine the relationship between Kerr rotation and spin accumulation in Cu by comparing the experiment with the model: we find rad m A −1 . Kerr rotation in NMs in an external magnetic field has been reported previously [41] , [42] ; a magnetic field produces spin accumulation in a NM by splitting energy of spin sub-bands. However, Kerr rotation in an applied field has an additional contribution from field-dependent scattering. As we measure the spin accumulation in Cu without an applied magnetic field, the field-dependent scattering term is absent and our measurement is only sensitive to spin accumulation. STT in the CoFeB layer The demagnetization-induced spin current discussed above has a spin component collinear with the [Co/Pt] magnetization. For the CoFeB-2 nm sample, therefore, this spin current is transverse to the CoFeB magnetization and could efficiently supply STT. The CoFeB layer acts as a spin sink due to a rapid dephasing of the transverse spin component within a few atomic layers of a FM [29] . The absorption of the transverse spin current by the CoFeB layer produces a tilting of its magnetization followed by precession. The most salient feature observed with the CoFeB-2 nm sample is that the precession of the CoFeB layer appears on top of the smooth background created by the demagnetization and magnetization recovery of the [Co/Pt] layer ( Fig. 5a ). (The Cu layer in this sample is thin, only 10 nm, and therefore the magneto-optic properties of the [Co/Pt] directly effects the polarization of the probe.) Spin current from the [Co/Pt] layer tilts the CoFeB-magnetization—which initially lies in-plane—out-of-plane within a few picoseconds; the CoFeB magnetization subsequently precesses. The initial tilting of CoFeB produces a positive Kerr rotation, while the demagnetization of [Co/Pt] produces a negative rotation. As the static Kerr rotations of CoFeB and [Co/Pt] are of the same sign, the direction of the initial CoFeB tilting is the same as that of the [Co/Pt] magnetization. The demagnetization-induced spin current should tilt the CoFeB magnetization to the direction of the Co/Pt magnetization, but the temperature gradient-induced spin current should tilt the CoFeB magnetization to the opposite direction (see Fig. 4b ). Therefore, we conclude that the demagnetization is more dominant than the temperature gradient. We discuss other possible origins for precession of the CoFeB magnetization and the possibility of [Co/Pt]-precession in Supplementary Note 6 and Supplementary Fig. 3 . 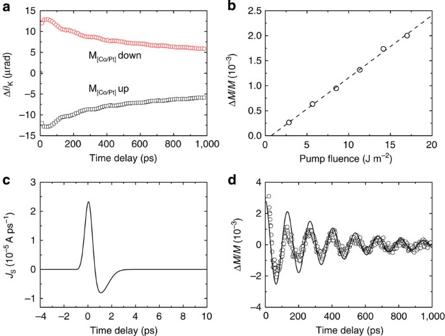Figure 5: STT on the CoFeB layer. (a) Kerr rotation of the CoFeB-2 nm sample with pump fluence of 17 J m−2with the [Co/Pt] magnetization up (black square) or down (red circle). (b) The normalized precession amplitude, ΔM/M, of the CoFeB with different pump fluence up to 17 J m−2(black circle). The dotted line is the linear fitting of data. (c) The calculated spin current that goes to CoFeB in the CoFeB-2 nm sample. The calculation is done by the spin diffusion simulation. (d) The precession data and magnetization dynamics simulation. The precession data (black circle) is obtained by subtracting the demagnetization signal ofaat the [Co/Pt] magnetization up. The magnetization dynamics simulation (black solid line) is done by Landau–Lifshitz–Gilbert equation with an input spin current ofc. Figure 5: STT on the CoFeB layer. ( a ) Kerr rotation of the CoFeB-2 nm sample with pump fluence of 17 J m −2 with the [Co/Pt] magnetization up (black square) or down (red circle). ( b ) The normalized precession amplitude, Δ M / M , of the CoFeB with different pump fluence up to 17 J m −2 (black circle). The dotted line is the linear fitting of data. ( c ) The calculated spin current that goes to CoFeB in the CoFeB-2 nm sample. The calculation is done by the spin diffusion simulation. ( d ) The precession data and magnetization dynamics simulation. The precession data (black circle) is obtained by subtracting the demagnetization signal of a at the [Co/Pt] magnetization up. The magnetization dynamics simulation (black solid line) is done by Landau–Lifshitz–Gilbert equation with an input spin current of c . Full size image After subtracting the demagnetization signal, the precession signal is well described by a damped sine function whose frequency, 7.4 GHz, and damping constant, 0.018, are can be calculated from the properties of CoFeB (see Supplementary Note 7 and Supplementary Fig. 4 ). The oscillation amplitude is 0.45±0.5 μrad at a pump fluence of 17 J m −2 . Comparing with the static Kerr rotation, 240±50 μrad, of the full magnetization of the CoFeB layer, the oscillation amplitude corresponds to . The precession amplitude of CoFeB is linearly proportional to the pump fluence and approach zero at zero pump fluence ( Fig. 5b ). This result is characteristic of the transverse STT. For collinear STT, where two magnetizations lie parallel or antiparallel, there should be a threshold of spin current to trigger a precession [4] . However, for the transverse STT, there should be no threshold, and the precession amplitude should go smoothly to zero at zero spin current, in agreement with our observations. We also observe that the precession amplitude of CoFeB decreases as the angle between [Co/Pt] and CoFeB deviates from transverse configuration (see Supplementary Note 8 and Supplementary Fig. 5 ). We compare the spin gain of the CoFeB layer and the spin loss of the [Co/Pt] layer. For the CoFeB layer, we calculate the spin gain as 4.8 × 10 −6 A by multiplying M S (=1.2 × 10 6 A m −1 ), thickness (=2 × 10 −9 m) and . For the [Co/Pt] layer, the spin loss by demagnetization is 7.8 × 10 −5 A, calculated in the same manner by multiplying M S (=4 × 10 5 A m −1 ), thickness (=6.5 × 10 −9 m) and . Thus, 6% of the spin loss of the [Co/Pt] layer is converted to the spin gain of the CoFeB layer. For a more quantitative estimate of the spin transfer, we solve the spin diffusion equation for the four-layer Pt/[Co/Pt]/Cu/CoFeB structure with the diffusion constant and relaxation time of each layer as described above. We set μ s =0 in the CoFeB layer as the CoFeB layer acts as a spin sink. We also include finite spin conductances at NM–FM interfaces [43] , [44] , because the interfacial spin conductance becomes dominant over the bulk diffusivity at thin Cu thickness. For the longitudinal component, the spin conductance is , and for the transverse component the spin conductance is , where G ↑ is the conductance of the majority spin, G ↓ is that of the minority spin and G ↑↓ is the spin mixing conductance [44] . As the spin in Cu and Pt is collinear with the [Co/Pt] magnetization and transverse with the CoFeB magnetization, we incorporate the longitudinal spin conductance in the model at the Pt/[Co/Pt] and [Co/Pt]/Cu interfaces, and the transverse spin conductance at the Cu/CoFeB interface. We use values for the spin conductances from the first-principles calculation of the Co/Cu interface [45] , G ↑ =0.42, G ↓ =0.33 and Re{ G ↑↓ }=0.56 × 10 15 Ω −1 m −2 . Performing spin diffusion simulation with these parameters, we determine the spin current that goes to CoFeB ( Fig. 5c ). Owing to the small spin relaxation time of [Co/Pt] and finite spin conductances at interfaces, only 9% of total spin generation by dM/dt of [Co/Pt] goes to CoFeB. Using the obtained J S as an input, we perform magnetization dynamics simulation for CoFeB with the Landau–Lifshitz–Gilbert equation incorporating STT [46] , [47] , [48] , where m and m fixed are unit vectors in the direction of the CoFeB and [Co/Pt] magnetizations, respectively, is the time derivative of m , M S and h are the saturation magnetization and thickness of the CoFeB layer, respectively, H eff is the effective field due to applied field and shape anisotropy of CoFeB, γ is the gyromagnetic ratio, α is the Gilbert damping constant and J S is the spin current. We use the same values for applied field, shape anisotropy and α of CoFeB as in Supplementary Note 7 . The simulation result is in good agreement with the precession data ( Fig. 5d ). The precession amplitude of the simulation is higher than that of the measurement, but considering uncertainties in the spin relaxation times, interfacial spin conductances and measurements, the agreement between data and simulation is good. Our models explain the experimentally observed spin current generation within the context of temperature differences between thermal reservoirs and temperature differences between different locations in the sample, that is, we successfully describe the spin current generation in terms of deviations from thermodynamic equilibrium. Electron–magnon coupling and differences in the temperatures of electrons and magnons in a rapidly heated ferromagnetic layer converts demagnetization to spin generation in the FM. The generated spin leads to spin accumulation in an adjacent NM and STT in a second ferromagnetic layer by diffusive spin transport. The demagnetization-induced STT occurs on picosecond timescales that are extremely challenging to achieve in electrical measurements. Thus, we refer to this spin current as thermally driven and believe that our results extend the emerging discipline of spin caloritronics into the regime of picosecond timescales. Our study provides new insights on the physical mechanisms governing the interplay of spin and heat at the nanoscale and addresses the fundamental limits of ultrafast spintronic devices for data storage and information processing. Sample preparation and characterization To observe spin accumulation in Cu driven by laser heating, we use a film structure of sapphire substrate/Pt (30)/[Co (0.4)/Pt (1)] × 4 / Co (0.2)/Ni (0.4)/Co (0.2)/Cu (80)/MgO (10)/Al 2 O 3 (5), where the numerical values in parenthesis are the layer thickness in nanometres. This sample is prepared using a seven-target sputter deposition system with a base pressure of <5 × 10 −8 Torr at the Korea Institute of Science and Technology. The [Co/Pt] layer is a metallic FM with perpendicular magnetic anisotropy. We characterized the magnetic properties of the [Co/Pt] layer with a vibrating sample magnetometer; the saturation magnetization is 4 × 10 5 A m −1 , the coercivity is 0.1 T and the remanent magnetization is approximately the same as the saturation magnetization. We insert a thin Co/Ni layer between [Co/Pt] and Cu layers to minimize spin scattering by the Pt layer [5] . We chose a Cu layer as the spin accumulation layer because of its relatively long spin diffusion length [36] . MgO and Al 2 O 3 layers are deposited to protect the Cu layer from oxidation. The MgO layer is sputtered deposited in the same deposition chamber as the metal layers; the Al 2 O 3 layer is deposited in a separate deposition system. To observe STT, we use a sample incorporating a second magnetic layer with in-plane magnetization. This sample has the structure sapphire substrate/Pt (30)/[Co (0.4)/ Pt (1)] × 4 /Co (0.2)/Ni (0.4)/Co (0.2)/Cu (10)/CoFeB (2)/MgO (10)/Al 2 O 3 (5), prepared at the Korea Institute of Science and Technology. The saturation magnetization of the CoFeB layer of 1.4 × 10 6 A m −1 is determined with thermally oxidized Si substrate/CoFeB (45) sample. To fit the precession result of CoFeB-2 nm sample with damped sine function, we reduced M S of CoFeB to 1.2 × 10 6 A m −1 . We expect this reduction is due to thin thickness of the CoFeB layer. We prepared an additional set of samples with varying Cu thickness between 10 and 200 nm using a three-target sputter deposition system at the University of Illinois. The film structure is sapphire substrate/Pt (30)/[Co (0.5)/ Pt (1)] × 4 /Co (0.5)/Cu ( h )/SiO 2 (10), where h denotes the Cu thickness 10< h <200 nm. We could not include the Ni layer in these structures because of the limitation on the number of targets. The SiO 2 layer is prepared by e-beam evaporator in a separate deposition system. Pump–probe measurement The wavelengths of the pump and probe pulses are centred at 785 nm and have a FWHM) spectral range of ∼ 10 nm. The 1/ e 2 intensity radius of the focused pump and probe are 5 μm. Pump optical pulses are incident on the Pt side of the samples through the sapphire substrate. As the pump pulses pass through an electro-optic modulator with a relatively large group-delay-dispersion, the FWHM duration of the pump pulses is relatively long, ∼ 0.8 ps. The FWHM duration of the probe pulses is ∼ 0.35 ps. We use TR-MOKE to detect the transient magnetic properties. The incident probe is linearly polarized; the rotation of the polarization on reflection from the surface of the sample is measured by splitting the probe beam with a Wollaston prism and detecting the changes in the intensity of the orthogonal polarization states using a balanced detector. The changes in the light intensity convert to the voltage signal after the balanced detector. We obtain the Kerr rotation from the voltage signal using a measured conversion factor between the voltage and rotation. We use a double modulation technique with the pump beam modulated at 10.7 MHz and the probe beam modulated at 200 Hz to further improve the signal-to-noise ratio and suppress background created by a diffusely scattered pump light. We set the zero time delay to the midpoint of the initial rise of the TDTR signal generated by Pt. Except for the precession measurement where we apply an external magnetic field of 0.045 T in the in-plane direction, all the measurements are conducted without an applied magnetic field. How to cite this article: Choi, G.-M. et al. Spin current generated by thermally driven ultrafast demagnetization. Nat. Commun. 5:4334 doi: 10.1038/ncomms5334 (2014).